AmiA is a penicillin target enzyme with dual activity in the intracellular pathogenChlamydia pneumoniae Intracellular Chlamydiaceae do not need to resist osmotic challenges and a functional cell wall was not detected in these pathogens. Nevertheless, a recent study revealed evidence for circular peptidoglycan-like structures in Chlamydiaceae and penicillin inhibits cytokinesis, a phenomenon known as the chlamydial anomaly. Here, by characterizing a cell wall precursor-processing enzyme, we provide insights into the mechanisms underlying this mystery. We show that AmiA from Chlamydia pneumoniae separates daughter cells in an Escherichia coli amidase mutant. Contrary to homologues from free-living bacteria, chlamydial AmiA uses lipid II as a substrate and has dual activity, acting as an amidase and a carboxypeptidase. The latter function is penicillin sensitive and assigned to a penicillin-binding protein motif. Consistent with the lack of a regulatory domain in AmiA, chlamydial CPn0902, annotated as NlpD, is a carboxypeptidase, rather than an amidase activator, which is the case for E. coli NlpD. Functional conservation of AmiA implicates a role in cytokinesis and host response modulation. C hlamydiaceae are characterized by an obligate intracellular lifestyle and a unique biphasic developmental cycle. Despite the economic and public health importance of ocular, respiratory and sexually transmitted diseases caused by Chlamydiaceae , our knowledge about their biology at a molecular level is still limited. One crucial aspect of chlamydial biology that remains to be elucidated is the long known, yet still enigmatic chlamydial anomaly: for endobacteria such as Chlamydiaceae , there is no need to maintain osmotic stabilization by means of a cell wall, and a functional cell wall has not been detected in these pathogens [1] . Nevertheless, antibiotics that target cell wall biosynthesis are active against Chlamydiaceae [1] . Penicillin has no bactericidal effect on Chlamydiaceae but induces a reversible state of persistence, a phenomenon that is observed during chronic, recurring infections with Chlamydia trachomatis and C. pneumoniae [2] . The bacterial mesh-like cell wall consists of peptidoglycan (PG), a polymer of sugar chains that are cross-linked via flexible peptide bridges. PG is evolutionary conserved in eubacteria with the exception of some obligate intracellular species. Biosynthesis of PG takes place in three compartments of bacterial cells [3] . In the cytoplasm, formation of the soluble precursors UDP- N -acetylglucosamine and UDP- N -acetylmuramyl-pentapeptide is catalysed. At the inner leaflet of the cytoplasmic membrane, the two precursors are assembled with the lipid carrier bactoprenol-phosphate (undecaprenyl-P) to form lipid II, the completed cell wall-building block. Lipid II is then translocated to the outside of the cell and incorporated into the PG network releasing undecaprenyl-PP. Prokaryotic cell division is driven by >10 essential proteins, which assemble at the septum to form the divisome [3] , [4] , [5] . Briefly, the following stages of cell division are recognized in E. coli : the tubulin orthologue FtsZ forms a ring-like structure (Z ring) at midcell and initiates divisome assembly by attracting a set of ‘early’ proteins to form a cytoplasmic apparatus linked to the membrane; then enzymes for lipid II biosynthesis and presumably for PG biosynthesis localize to the midcell to carry out ‘preseptal’ elongation, a process in which the actin orthologue MreB might participate; additional elements co-ordinate chromosome segregation and build an extracellular connector for outer membrane constriction; finally, proteins involved in the incorporation (for example, transpeptidase FtsI (penicillin-binding protein (PBP) 3) and flippase FtsW) and remodelling (amidases) of septal PG assemble. The process ends with cell segregation. The three periplasmic N -acetylmuramyl- L -alanine amidases AmiA, AmiB and AmiC have been shown to be important for cell separation in E. coli . Double- and triple-amidase mutants form cell chains to varying extents [6] , [7] . The chain-forming amidase mutants constrict the inner membrane, fail to split septal PG, are connected by shared PG layers and partially constrict their outer membranes [6] , [7] . In contrast to AmiB and AmiC, AmiA is not localized to the septum [3] . Nevertheless, E. coli double mutants with only AmiA are still able to partially separate [6] . AmiA, AmiB and AmiC are members of the zinc-dependent N -acetylmuramyl- L -Ala amidase 3 family and catalyse the release of peptide moieties from PG by cleaving the amide bond between the lactyl group of muramic acid and the amino group of L -alanine. In E. coli the amidases AmiA, AmiB and AmiC need to be activated by LytM domain proteins to efficiently hydrolyse septal PG. EnvC has been shown to serve as a specific activator for AmiA and AmiB, and NlpD specifically activates AmiC [8] . In previous studies, E. coli AmiA has been shown to hydrolyse polymeric PG [8] , as well as glycan strands of varying chain length consisting of at least two transglycosylated lipid II cell wall-building blocks in a zinc-dependent fashion in vitro . Monomeric lipid II was not degraded by E. coli AmiA, suggesting that the enzyme requires at least a tetrasaccharide as a substrate [9] . Despite massive reduction in the genome size, a nearly complete pathway for lipid II biosynthesis has been found in Chlamydiaceae genomes [1] , and activity of enzymes catalysing cytoplasmic steps (MurA, MurC/Ddl, CT390, DapF, MurE, GlyA and MurF) and the two membrane-linked steps (MraY and MurG) of cell wall precursor synthesis has been demonstrated [1] , [10] , [11] , [12] , [13] , [14] . Chlamydiaceae genomes retained two periplasmic enzymes that are involved in side-wall (PBP2) and septal (FtsI (PBP3)) incorporation of lipid II building blocks in free-living rod-shaped bacteria such as E. coli . Moreover, the human pathogens harbour a rudimentary set of divisome proteins, lacking the almost ubiquitous central organizer FtsZ, but including FtsW, FtsI (PBP3) and FtsK, and possess, despite their spherical shape, the cytoskeletal protein MreB [1] , [15] . AmiA is the only amidase encoded by Chlamydiaceae genomes and cell wall remodelling enzymes such as endopeptidases and lytic transglycosylases have not been identified [1] . We discussed that maintaining biosynthesis of the cell wall-building block lipid II in cell wall-lacking ‘minimal bacteria’ such as Chlamydiaceae may reflect a vital role of the lipid II pathway in prokaryotic cell division [13] . Moreover, we proposed that MreB is involved in orchestration of lipid II biosynthesis at the septum and as such may be necessary for maintaining a functional divisome machinery in Chlamydiaceae [15] . Recently, a cell wall sacculus was detected in the evolutionary earlier, genomically less reduced environmental chlamydiae Protochlamydia [16] . However, consistent with our model described above, MreB and its interacting partner RodZ from the environmental chlamydial genus Waddlia have been shown to localize to the septum [17] , and in Chlamydiaceae no cell wall but a distinct circularly shaped structure was found. This structure was suggested to consist of rudimentary PG-like material that is localized to the septum of dividing cells [18] . The aim of this study was to gain first mechanistic insights in processing of chlamydial lipid II at the division site. Here, we demonstrate that amidase AmiA is functionally conserved in Chlamydiaceae and capable of using the monomeric cell wall-building block lipid II as a substrate for amidase and novel penicillin-sensitive DD-carboxypeptidase (DD-CPase) activity in vitro . AmiA-driven processing of lipid II might be crucial for a complete lipid II biosynthesis and recycling cycle, and thus for maintaining coordinated cell division in Chlamydiaceae . Moreover, lipid II processing might modulate host response to muropeptides. AmiA from C. pneumoniae is functional in E. coli AmiA from C. pneumoniae (AmiA Cp ) and E. coli show 32% amino-acid sequence identity. If AmiA Cp is capable of degrading PG, as shown before for the homologue of E. coli [8] , the enzyme might lyse bacterial cells. Overexpression of AmiA Cp in the periplasm of E. coli was achieved by fusion to the OmpA leader peptide and resulted in lysis of the producer strain after induction ( Fig. 1a ). To investigate functionality of AmiA Cp in cell separation of free-living bacteria, we performed complementation assays using an E. coli ΔamiABC triple-knockout mutant harbouring an arabinose-inducible amiC gene on a plasmid ( Fig. 1b ). When grown in the presence of glucose, the cells fail to separate during cell division and form long chains ( Fig. 1c ). The expression of AmiA Cp resulted in separated rod-shaped cells ( Fig. 1c ). Quantitative analysis of the experiments revealed that virtually all cells of the amidase triple mutant were present in chains ( Fig. 1d ). Upon induction of AmiA Cp expression, the separation of daughter cells was rescued and 55% of the cells were single or paired ( Fig. 1d ). These data are in agreement with 30–40% chains observed in an E. coli ΔamiBΔamiC mutant containing AmiA [6] . In total, these findings indicate that AmiA Cp can perform daughter cell separation in E. coli , presumably by the degradation of septal PG during cell division. 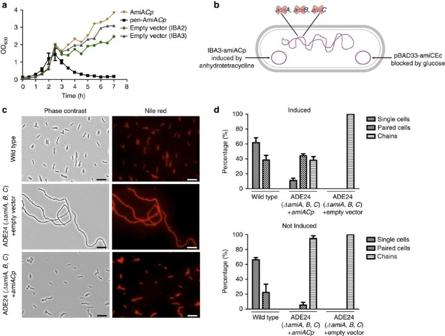Figure 1: Activity of AmiACpinE. coli. Growth kinetics ofE. colJM83 containing chlamydialamiAconstructs. (a) AmiA expression was induced at an OD600of 0.6. Periplasmic expression of AmiACp(peri-AmiACp) resulted in lysis ofE. coliJM83. Without being fused to the OmpA leader peptide (AmiACp), AmiA did not accumulate sufficiently at the periplasm to cause lysis of the expression strain. Error bars indicate±s.d. (n=3). Complementation ofE. coli ΔamiABCtriple-knockout mutant ADE24 by chlamydial AmiA (b–d). Illustration ofE. coliADE24 (b). The mutant was transformed with plasmid IBA3-amiACp that allows for AHT-induced expression of AmiACp; microscopy (c) and quantative (d) analyses of the experiments: in the presence of glucose and AHT, expression of AmiC fromE. coliwas blocked and complementation of the chain-forming triple-amidase mutant by AmiACpresulted in separated rod-shaped cells. Error bars are mean±s.d. (n=3). Scale bar, 10 μm. A control experiment with AmiA fromE. coliis presented inSupplementary Fig. 5. Figure 1: Activity of AmiA Cp in E. coli . Growth kinetics of E. col JM83 containing chlamydial amiA constructs. ( a ) AmiA expression was induced at an OD 600 of 0.6. Periplasmic expression of AmiA Cp (peri-AmiA Cp ) resulted in lysis of E. coli JM83. Without being fused to the OmpA leader peptide (AmiA Cp ), AmiA did not accumulate sufficiently at the periplasm to cause lysis of the expression strain. Error bars indicate±s.d. ( n =3). Complementation of E. coli ΔamiABC triple-knockout mutant ADE24 by chlamydial AmiA ( b – d ). Illustration of E. coli ADE24 ( b ). The mutant was transformed with plasmid IBA3-amiACp that allows for AHT-induced expression of AmiA Cp ; microscopy ( c ) and quantative ( d ) analyses of the experiments: in the presence of glucose and AHT, expression of AmiC from E. coli was blocked and complementation of the chain-forming triple-amidase mutant by AmiA Cp resulted in separated rod-shaped cells. Error bars are mean±s.d. ( n =3). Scale bar, 10 μm. A control experiment with AmiA from E. coli is presented in Supplementary Fig. 5 . Full size image AmiA Cp shows amidase activity on the PG and lipid II precursor Purified AmiA Cp was tested for degradation of PG using a remazol dye-release assay. As shown before for E. coli amidases [8] , AmiA Cp released remazol-stained reaction products into the supernatant from the PG sacculi ( Fig. 2a,b ). A control protein (DD-CPase VanY) that removes D -Ala from the peptide side chains, did not release the dye. 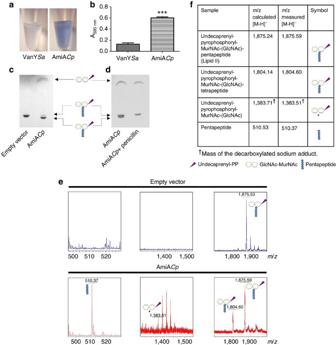Figure 2:In vitroactivity of AmiACp. The enzyme used PG as well as monomeric lipid II as a substrate. Dye-release assay on the degradation of PG: released reaction products after incubation of remazol-stained PG with control enzyme VanY fromStaphylococcus aureus(VanYSa) and AmiACp(a) and photometric analysis of supernatants (b). Error bars indicate±s.d. (n=3). Unpairedt-test revealed statistical significance in comparision with VanY control, two-tailed ***P-value ≤0.0001. TLC analysis (c,d) and MS (e,f) of lipid II reaction products. AmiACpshowed novel amidase and DD-CPase activity on lipid II. The latter function was sensitive to penicillin. *The O-1-carboxyethyl-residue at position 3 in the MurNAc moiety of the amidase reaction product undecaprenyl-pyrophosphoryl-MurNAc-GlcNAc is decarboxylated, as usually observed with the matrix 6-Aza-2-thiothymine46. Additional peaks in the spectrum for the decarboxylated undecaprenyl-pyrophosphoryl-MurNAc-GlcNAc sodium adduct are attributed to the addition of water to conjugated double bonds in the undecaprenyl moiety (mass shift of 18 Da). (GlcNAc: N-acetylglucosamine; MurNAc: N-acetylmuramic acid). Figure 2: In vitro activity of AmiA Cp . The enzyme used PG as well as monomeric lipid II as a substrate. Dye-release assay on the degradation of PG: released reaction products after incubation of remazol-stained PG with control enzyme VanY from Staphylococcus aureus (VanY Sa ) and AmiA Cp ( a ) and photometric analysis of supernatants ( b ). Error bars indicate±s.d. ( n =3). Unpaired t -test revealed statistical significance in comparision with VanY control, two-tailed *** P -value ≤0.0001. TLC analysis ( c , d ) and MS ( e , f ) of lipid II reaction products. AmiA Cp showed novel amidase and DD-CPase activity on lipid II. The latter function was sensitive to penicillin. *The O-1-carboxyethyl-residue at position 3 in the MurNAc moiety of the amidase reaction product undecaprenyl-pyrophosphoryl-MurNAc-GlcNAc is decarboxylated, as usually observed with the matrix 6-Aza-2-thiothymine [46] . Additional peaks in the spectrum for the decarboxylated undecaprenyl-pyrophosphoryl-MurNAc-GlcNAc sodium adduct are attributed to the addition of water to conjugated double bonds in the undecaprenyl moiety (mass shift of 18 Da). (GlcNAc: N-acetylglucosamine; MurNAc: N-acetylmuramic acid). Full size image Chlamydiaceae do not contain detectable quantities of PG but retained the biosynthesis pathway of the cell wall-building block lipid II [13] . We tested whether chlamydial AmiA can remove the pentapeptide side chain from the membrane-bound cell wall precursor. Thin-layer chromatography (TLC) analysis of lipid II reaction products combined with mass spectrometry (MS) revealed that AmiA Cp was capable of using lipid II as a substrate for amidase activity and cleaved the peptide side chain from the sugar moieties of lipid II ( Fig. 2c–f ). In summary, AmiA Cp is an N -acetylmuramyl- L -alanine amidase using polymeric PG and monomeric lipid II as a substrate in vitro . AmiA Cp has an additional function as DD-CPase Surprisingly, our TLC/MS analysis showed that chlamydial AmiA exhibited dual enzymatic activity on lipid II in vitro . In addition to the amidase product, we identified lipid II with a tetrapeptide, indicating that cleavage of the terminal D -Ala residues had occurred ( Fig. 2c–f ). Therefore, AmiA has also DD-CPase activity. It was possible that the heterologous AmiA produced in E. coli was contaminated by host DD-CPases (class C PBPs). To test this possibility, we performed several control experiments. A mock protein purification from the E. coli strain harbouring the empty vector had no detectable DD-CPase activity ( Fig. 2c ) and we did not detect any PBPs in the AmiA Cp preparation when labelling with fluorescent penicillin bocillin FL ( Supplementary Fig. 1 ), making it unlikely that the DD-CPase detected was due to contaminating host PBPs. The enzyme had no beta-lactamase activity in a nitrocefin hydrolysis-based test system ( Supplementary Fig. 2 ), indicating that the detection of possibly contaminating PBPs was not impaired by hydrolysis of bocillin FL. Of note, DD-CPase activity of AmiA Cp was sensitive to penicillin and blocked in a molar ratio of 1:1 (protein:inhibitor), whereas amidase activity was not impaired in the presence of the beta-lactam ( Fig. 2d ; Supplementary Fig. 3 ). Our results identify AmiA Cp as a novel DD-CPase and, besides PBP2, PBP3 and PBP6, as an additional so far unknown target of beta-lactams in Chlamydiaceae. Inactivation of the amidase active site The active site of E. coli AmiA is comprised by three zinc coordinating residues (H65, E80 and H133) and E242 that is predicted to serve as a general base catalyst [9] . We found all residues to be conserved in AmiA Cp ( Fig. 3 ) and replaced H67, H136 and E207 (corresponding to H65, H133 and E242 in E. coli ) with alanine to explore their functional role in amidase activity. Expression of AmiAH67A Cp and AmiAH136A Cp mutants at the periplasm impaired growth of the E. coli expression strain but did not lead to cell lysis ( Fig. 4a ). The exchange of E207 had no effect on the lytic activity of AmiA Cp . These results indicate that both histidine residues are essential for amidase activity of AmiA Cp , as shown before for the corresponding residues in E. coli [9] . In contrast, the glutamic acid, which is necessary for AmiA activity in E. coli [9] , is not needed for amidase function in the chlamydial homologue. We further investigated whether inactivation of the amidase active site affects DD-CPase activity. The AmiAH67ACp mutant was still capable of cleaving terminal D -Ala residues from the pentapetide side chain of lipid II, implicating that both activities are independent from each other ( Supplementary Fig. 4a ). 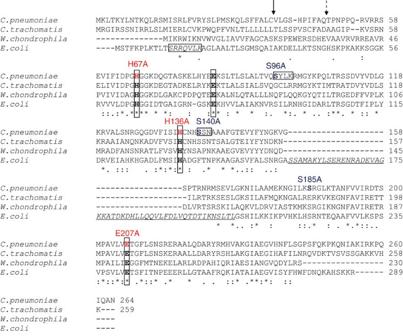Figure 3: Sequence alignment of AmiA fromE. coliand selectedChlamydialesspecies. The amidase active site ofE. coliAmiA contains three zinc-coordinating residues (H65, E80 and H133), and E242 that is predicted to serve as a general base catalyst9. These active site residues (in bold and boxed) are highly conserved in theChlamydialesspecies. Of note, theChlamydialesAmiA proteins lack a domain with predicted autoregulatory functions (underlined and in italics) that is exclusively found in cell division amidases AmiA, AmiB and AmiC and contains an α-helix (S157-V173 inE. coliAmiA, corresponding to D280-L296 in AmiB fromB. henselae) occluding the active site. During cell division, the regulatory domain is proposed to interact with LytM domain factors to relieve autoinhibition by a conformational switch25. PBP DD-CPases have three typical motifs, SxxK, S(Y)xN and K(H,R)T(S)G, that are essential for substrate recognition and catalysis. AmiA fromC. pneumoniaecontains an SxxK and an SxN motif but lacks the KTG motif. The signal peptide fromE. colicontains an SRRxFLK (with x being a polar amino acid) consensus motif (boxed and in italics) that directs AmiA to the Tat translocation system. Consistent with the absence of a Tat system in chlamydiae, AmiA fromC. pneumoniaedoes not contain a functional Tat motif. The solid arrow and the dashed arrow point to the signal peptidase cleavage sites in AmiA fromC. pneumoniaerevealed by MS analysis and predicted by SignalP32, respectively. Figure 3: Sequence alignment of AmiA from E. coli and selected Chlamydiales species. The amidase active site of E. coli AmiA contains three zinc-coordinating residues (H65, E80 and H133), and E242 that is predicted to serve as a general base catalyst [9] . These active site residues (in bold and boxed) are highly conserved in the Chlamydiales species. Of note, the Chlamydiales AmiA proteins lack a domain with predicted autoregulatory functions (underlined and in italics) that is exclusively found in cell division amidases AmiA, AmiB and AmiC and contains an α-helix (S157-V173 in E. coli AmiA, corresponding to D280-L296 in AmiB from B. henselae ) occluding the active site. During cell division, the regulatory domain is proposed to interact with LytM domain factors to relieve autoinhibition by a conformational switch [25] . PBP DD-CPases have three typical motifs, SxxK, S(Y)xN and K(H,R)T(S)G, that are essential for substrate recognition and catalysis. AmiA from C. pneumoniae contains an SxxK and an SxN motif but lacks the KTG motif. The signal peptide from E. coli contains an SRRxFLK (with x being a polar amino acid) consensus motif (boxed and in italics) that directs AmiA to the Tat translocation system. Consistent with the absence of a Tat system in chlamydiae, AmiA from C. pneumoniae does not contain a functional Tat motif. The solid arrow and the dashed arrow point to the signal peptidase cleavage sites in AmiA from C. pneumoniae revealed by MS analysis and predicted by SignalP [32] , respectively. 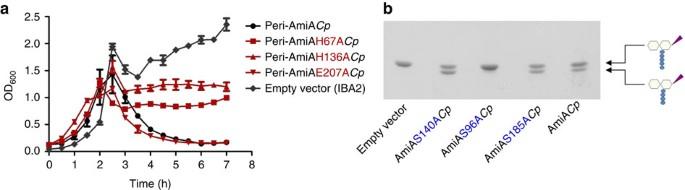Figure 4: Characterization of active sites. Studies of the amidase active site (a). The zinc-coordinating His residues are essential for the lytic activity of AmiACp. Error bars indicate±s.d. (n=3). Discovery of the amino acids involved in DD-CPase activity (b). The exchange of residue S96 in the SxxK tetrad leads to a loss of function. Full size image Figure 4: Characterization of active sites. Studies of the amidase active site ( a ). The zinc-coordinating His residues are essential for the lytic activity of AmiA Cp . Error bars indicate±s.d. ( n =3). Discovery of the amino acids involved in DD-CPase activity ( b ). The exchange of residue S96 in the SxxK tetrad leads to a loss of function. Full size image Identification of the DD-CPase active site Penicillin-sensitive PBP DD-CPases, including VanY D DD-CPase from vancomycin-resistant Enterococcus faecium [19] , are acyl-serine transferases and contain three typical motifs, SxxK, S(Y)xN and K(H,R)T(S)G, that are essential for substrate recognition and catalysis [20] . AmiA Cp has an SxxK (S96-Y97-L98-K99) and an SxN motif (S140-S141-N142), but no KTG motif ( Fig. 3 ). The zinc-dependent DD-CPase of Streptomyces albus as well as PdcA from Myxococcus xanthus [20] and VanY [21] and VanY B [22] from enterococci are DD-CPases that are beta-lactam insensitive. AmiA Cp has neither the zinc-binding motif H(x42aa)HxH of the S. albus enzyme [23] nor the motifs SxHxxGxA(S)xD and EP(W)WH conserved in the DD-CPases VanY , VanYB and PdcA [20] , [24] . Recently, the first structure of a cell separation amidase, AmiB from Bartonella henselae , was solved [25] . We conducted a search for similar structures to AmiB from B. henselae using the DALI server [26] and found matches with members of the carboxypeptidase A family ( Z -scores ranging from 9.8–8). This zinc metalloprotease family is dominated by mammalian enzymes but comprises a few proteins of bacterial origin such as the γ- D -glutamyl-( L )-mDAP-hydrolysing peptidase I from Bacillus sphaericus [27] . To identify amino acids that are involved in the DD-CPase function of AmiA Cp , we replaced the serine residues S96 and S140 in the two PBP homologous motifs SxxK and SxN as well as the residue S185, which is conserved in AmiA from E. coli and Chlamydiaceae and found in peptidase I from B. sphaericus . The replacement of S96 abolished DD-CPase activity, whereas the other mutations had no effect ( Fig. 4b ). These results provide further proof that the observed activity was not owing to a contaminating host PBP in the purified protein. The penicillin-sensitive DD-CPase function seems to be conferred solely by an SxxK motif independently from the apparently not essential SxN triad and the absent KTG motif. This is different from conventional bacterial PBPs whose activity depend, in addition to the SxxK tetrad, on a functional SxN motif and which typically contain a KTG motif as well [28] . The DD-CPase active site mutant AmiAS96A Cp was not impaired in amidase activity, providing further evidence that both enzymatic activites of AmiA Cp are independent from each other ( Supplementary Fig. 4b ). Secretion of AmiA Cp AmiA from E. coli contains a twin-arginine translocation (Tat) motif and is transported to the periplasm by the Tat system [29] . Consistent with the absence of a Tat system in Chlamydiaceae , AmiA Cp does not have an SRRxFLK Tat consensus motif ( Fig. 3 ) [30] , [31] , but contains a putative signal peptide. Without being fused to the OmpA leader peptide, the overexpressed AmiA Cp did not accumulate efficiently in the periplasm to lyse the E. coli producer strain ( Fig. 1a , AmiA Cp ). Nevertheless, in the complementation assay, native AmiA Cp was able to rescue cell separation in the E. coli amidase triple mutant ( Fig. 1c,d ), whereas AmiAΔSP Cp , which lacks the putative signal peptide, failed to complement the mutant ( Supplementary Fig. 5 ). MS of the heterologously expressed native AmiA Cp revealed cleavage of the signal peptide in E. coli between residues 37 and 38 and not further downstream as frequently found for Tat signal peptides and predicted by SignalP ( Fig. 3 ) [32] . Thus, our data indicate that AmiA Cp contains a functional Sec signal peptide. Chlamydial AmiA lacks an autoregulatory domain The active sites of the cell division amidases AmiA, AmiB and AmiC from Gram-negative bacteria are likely to be occluded by a conserved α-helix, as previously shown for AmiB from B. henselae [25] . These amidases have low basal in vitro activity and need to be activated by EnvC or NlpD. The LytM-containing septal ring factors are thought to specifically interact with the autoregulatory domain of the corresponding enzymes (EnvC with AmiA and AmiB and NlpD with AmiC) to promote the release of the regulatory helix from the active site [25] . Sequence analysis showed that AmiA Cp lacks this autoinhibitory domain (α-helix 5, aa 292–340 in E. coli AmiB, see alignment Fig. 3 ) and is unlikely to be autoregulated comparable to phage and mother cell lysis amidases such as CD27L, PLY-PSA and CwlVc [25] . The absence of an autoregulatory helix in AmiA Cp is consistent with the fact that Chlamydiaceae harbour neither the corresponding activator EnvC nor the AmiC activator NlpD. Moreover, the rudimentary divisome machinery of Chlamydiaceae lacks FtsE and FtsX, which have been shown to recruit the AmiA and AmiB activator EnvC to the septum in E. coli [33] . CPn0902, annotated as NlpD in C. pneumoniae , does not contain a LytM domain but two putative PG-binding LysM domains in the C-terminus. The companion paper by Frandi et al. [34] demonstrates that expression of Waddlia NlpD in E. coli increases the ratio of muro-tetrapeptide monomers to dimers in the PG. Consistently, purified Cpn0902 (NlpD) from C. pneumoniae was capable of releasing terminal D -Ala residues from the pentapeptide side chain of lipid II showing that the protein is rather a DD-CPase than an amidase-activating factor ( Fig. 5 ). 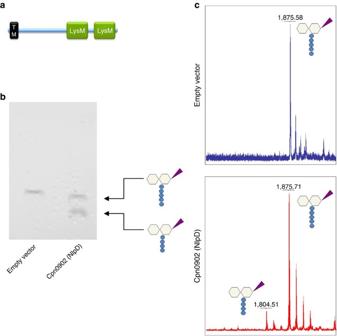Figure 5: Structure andin vitroactivity of Cpn0902 (NlpD). Conserved LysM (peptidoglycan-binding lysin subgroup) domains (identified using InterPro protein sequence analysis and classification tool, EMBL-EBI47) and a transmembrane domain (TM) are depicted (predicted by TMHMM software, Technical University of Denmark48) (a). TLC (b) and MS (c) analysis of reaction products revealed DD-CPase activity of Cpn0902 on lipid II. Figure 5: Structure and in vitro activity of Cpn0902 (NlpD). Conserved LysM (peptidoglycan-binding lysin subgroup) domains (identified using InterPro protein sequence analysis and classification tool, EMBL-EBI [47] ) and a transmembrane domain (TM) are depicted (predicted by TMHMM software, Technical University of Denmark [48] ) ( a ). TLC ( b ) and MS ( c ) analysis of reaction products revealed DD-CPase activity of Cpn0902 on lipid II. Full size image Since the first description of the chlamydial anomaly in 1993, several studies proved the functionality of early cytoplasmic steps [1] , [10] , [11] , [12] , [14] and of the two cytoplasm membrane-associated steps [13] of lipid II biosynthesis in Chlamydiaceae . This is the first description of a chlamydial lipid II-processing enzyme in the periplasm. In reticulate bodies, the replicative form of Chlamydiaceae , cell division is reversibly arrested by the second binary fission in the presence of penicillin, resulting in four enlarged, non-infectious bodies [35] . In free-living bacteria, the bactericidal effect of penicillin is owing to uncontrolled activity of PG hydrolases while PBP-conferred transpeptidase activity is blocked [36] . The genomes of Chlamydiaceae encode only one PG hydrolase, the cell division amidase AmiA. Uncontrolled AmiA activity does not lead to cell lysis in the isotonic niche and in the absence of a cell wall, making these ‘minimal bacteria’ an ideal tool to further analyse the action of beta-lactams beyond inhibition of PBP-catalysed transpeptidation and osmotic destabilization. Previously, a role of amidases in generating a glycan-less wall polypeptide was proposed for Chlamydiaceae [37] . We have previously discussed a model for co-ordination of the lipid II pathway and cell division in Chlamydiaceae [13] , [15] that implicates a central function of AmiA in sustaining an entire cycle of lipid II biosynthesis, processing and recycling ( Fig. 6 ): MreB (in interaction with RodZ) functionally organizes lipid II biosynthesis at the septum and the synthesized building block is processed by a rudimentary cell wall biosynthesis/cell division machinery. Following translocation to the periplasm, AmiA and monofunctional transpeptidases PBP2 and FtsI (PBP3) process the cell wall-building block in a concerted way to facilitate the release of the bactoprenol carrier. In this step, the rudimentary PG-like product found by Liechti et al. [18] in which the peptide side chains are cross-linked by peptide bonds might result. As our data show that AmiA Cp is also active against polymeric PG, we cannot rule out the possibility that the enzyme is involved in the turnover of the ring-like-shaped PG-like structure as well. The fate of the sugar units and turnover pathways for the cross-linked peptide side chains during the chlamydial developmental cycle are unknown. Moreover, recycling of bactoprenol-P remains unclear in the absence of pyrophoshorylases that have been described so far to dephosphorylate bactoprenol-PP [38] . 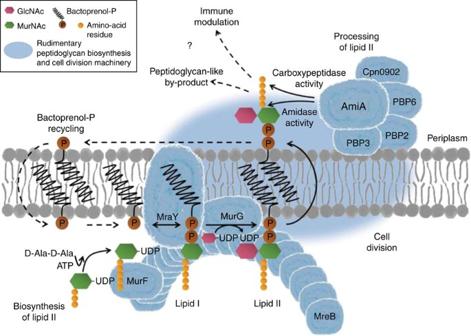Figure 6: Proposed model for the role of the conserved lipid II pathway in maintaining a functional cell division machinery and contributing to modulation of host response inChlamydiaceae. A complete cycle of lipid II biosynthesis, processing and recycling needs to be maintained for coordinated function of the cell division machinery. Structural protein MreB (in interaction with RodZ) functionally organizes MurF, MraY and MurG, three key components in lipid II biosynthesis, at the septum. The synthesized precursor is translocated to the outside and processed by a rudimentary cell wall biosynthesis/cell division machinery. DD-CPase activity of AmiA, together with PBP6 and Cpn0902 (NlpD), might orchestrate DD-CPase functions in chlamydial cell division. Amidase activity of AmiA would play a central role in processing lipid II by releasing the pentapeptide side chain to allow for (i) transpeptidation of pentapeptides catalysed by monofunctional transpeptidases FtsI and PBP2 and for (ii) regulation of host immune response due to blocking of Nod2 sensing. FtsZ as well as transglycosylases, endopeptidases and pyrophosphorylases are not found inChlamydiaceae. Dashed arrows and question marks indicate steps of the proposed pathway that remain to be elucidated. (GlcNAc:N-acetylglucosamine; MurNAc:N-acetylmuramic acid). Figure 6: Proposed model for the role of the conserved lipid II pathway in maintaining a functional cell division machinery and contributing to modulation of host response in Chlamydiaceae . A complete cycle of lipid II biosynthesis, processing and recycling needs to be maintained for coordinated function of the cell division machinery. Structural protein MreB (in interaction with RodZ) functionally organizes MurF, MraY and MurG, three key components in lipid II biosynthesis, at the septum. The synthesized precursor is translocated to the outside and processed by a rudimentary cell wall biosynthesis/cell division machinery. DD-CPase activity of AmiA, together with PBP6 and Cpn0902 (NlpD), might orchestrate DD-CPase functions in chlamydial cell division. Amidase activity of AmiA would play a central role in processing lipid II by releasing the pentapeptide side chain to allow for (i) transpeptidation of pentapeptides catalysed by monofunctional transpeptidases FtsI and PBP2 and for (ii) regulation of host immune response due to blocking of Nod2 sensing. FtsZ as well as transglycosylases, endopeptidases and pyrophosphorylases are not found in Chlamydiaceae . Dashed arrows and question marks indicate steps of the proposed pathway that remain to be elucidated. (GlcNAc: N -acetylglucosamine; MurNAc: N -acetylmuramic acid). Full size image According to our model, chlamydial AmiA would play a crucial role in processing lipid II in the periplasm. Consistent with the lack of a Tat system in Chlamydiaceae , our data indicate that AmiA is secreted across the cytoplasmic membrane by the Sec system. Moreover, we showed that AmiA is a functionally conserved amidase in Chlamydiaceae and is capable of using the monomeric building block lipid II as a substrate. Surprisingly, chlamydial AmiA did not only cleave the peptide side chain from the sugar moieties, but also exhibited DD-CPase activity on lipid II and released the terminal D -Ala from the peptide side chain in vitro . In accordance with the observed sensitivity to penicillin, we identified an SxxK motif to mediate the novel DD-CPase activity in the bifunctional enzyme. Sporulation protein SpoIIP from B. subtilis has been shown to exhibit amidase and endopeptidase activity [39] , whereas Atl-like staphylococcal autolysins are bifunctional enzymes with amidase and N -acetylglucosaminidase activity [40] , [41] . To our knowledge, AmiA Cp is the first example of an enzyme possessing amidase and DD-CPase activity. Moreover, our study revealed that AmiA is a so far unknown target of penicillin in Chlamydiaceae , besides the PBPs PBP2, PBP3 and PBP6. It is not known whether homologous amidases from E. coli and other free-living pathogens have a dual activity such as chlamydial AmiA. Recruitment to the division site might be conferred by interaction with PBPs. For both PBP3 and PBP2 from C. trachomatis , interactions with the cell division protein FtsK have been shown in bacterial two-hybrid experiments [42] . Many free-living bacteria have several low-molecular weight PBP DD-CPases, indicating an important but not completely understood physiological role for these peptidases. In E. coli the DD-CPase PBP5 is required for cell shape maintenance and proper division site placement, in particular, in mutants lacking other PG enzymes. Loss of PBP5 in a Δ amiC mutant enhances chain formation and the helical morphology of FtsZ inhibitor SulA-induced filaments is dependent on PBP5 (ref. 20) [20] . E. coli PBP6 has been implicated in stabilizing the stationary phase PG and in the function of the cell division-specific transpeptidase PBP3 (ref. 20) [20] . Chlamydiaceae have a single PBP DD-CPase homologous to E. coli PBP6. PBP6, AmiA and Cpn0902 (NlpD) might together provide DD-CPase functions for chlamydial cell division. Besides its role in cell division, the conserved lipid II pathway might contribute to sustaining long-term residence in infected cells and thus to pathogenicity. Induction of cytokines during chlamydial infections is not exclusively conferred by Toll-like receptor-dependent mechanisms or the adapter protein MyD88 signalling pathway [1] . Moreover, intracellular chlamydiae are recognized by human cytosolic pattern recognition receptors Nod1 and Nod2, which sense bacterial cell wall fragments to signal through a MyD88-independent pathway and mediate activation of the transcription factor NFκB [1] . The amidase activity provided by AmiA could be involved in host response regulation ( Fig. 6 ) comparable to eukaryotic PG recognition protein-L, which has amidase activity and may reduce host pro-inflammatory response to PG [43] . The concept of PG degradation as a common pathogenic strategy to subvert muropeptide recognition and host innate immunity has been described for other chronic human pathogens as well. Mycobacterium tuberculosis releases ‘stealth’ muropeptides catalysed by the resuscitation-promoting factors in concerted action with endopeptidase RipA or enzymes that modify pentapeptide side chains [43] . In Helicobacter pylori , AmiA activity blocks Nod2 sensing as this receptor is incapable of recognizing released peptide side chains disconnected from an intact N -acetylmuramic acid sugar unit [43] , [44] . Further studies on the processing machinery of lipid II in Chlamydiaceae are needed for a better understanding of the chlamydial anomaly and the functions of amidases in cell division. Moreover, deeper insights into immune modulation, long-term residence in infected cells and chlamydial persistence in patients will be achieved. Bacterial strains and growth conditions E. coli JM83 carrying AmiA expression plasmids and E. coli ADE24 were maintained on Luria Bertani (LB) agar plates containing 100 μg ml −1 ampicillin and 30 μg ml −1 chloramphenicol, respectively. Growth kinetics E. coli JM83 harbouring expression vectors was grown in LB and induced with 200 ng ml −1 anhydrotetracycline (AHT) at an OD 600 of 0.6. Construction of E. coli ADE24 E. coli MHD41 carries a markerless deletion in amiB [6] . We first deleted amiA by P1 transduction with JW2428 from the Keio E. coli mutant strain collection [45] , followed by the excision of the kanamycin resistance gene. Next, the amiC gene was deleted by P1 transduction with JW5449 from the Keio collection, followed by removal of the kanamycin resistance gene. The amiC gene was amplified by PCR from pBADAmiC [6] using the oligonucleotides SacIamiCup and HindIIIamiCdw ( Supplementary Table 1 ), which introduce Sac I and Hind III restriction sites upstream and downstream, respectively, of amiC . The amiC gene was then cloned in plasmid pBAD33 and the resulting pBAD33- amiCEc was transformed into the triple-amidase mutant to obtain strain ADE24. Cloning of amiA The amiA gene from C. pneumoniae GiD was amplified by PCR using the primers listed in Supplementary Table 1 and cloned into pASK-IBA2 and pASK-IBA3 using the Bsa I restriction site to generate an N-terminal OmpA-leader peptide fused, C-terminal Strep-tagged protein for periplasmic overproduction and a native signal peptide containing, C-terminal Strep-tagged protein for complementation assays, respectively. Site-directed mutagenesis H67, S96, H136, S140, S185 and E207 in AmiA Cp were changed to Ala using the QuikChange Lighting Site-Directed Mutagenesis Kit (Agilent Technologies, Germany). The respective sense and antisense primers listed in Supplementary Table 1 were used according to the manufacturer’s instructions. Correct base changes were confirmed by sequencing. In vivo complementation assay E. coli ADE24 harbours an E. coli amiC encoding pBAD33 vector and shows an inducible chain-forming phenotype in the presence of glucose ( Fig. 2 ; Supplementary Table 1 ). E. coli ADE24 was transformed with vector IBA3- amiACp allowing for expression of AmiA Cp including its native N-terminal signal peptide upon induction by AHT. Cells were grown in the same medium used for overproduction of AmiA Cp containing 30 μg ml −1 chloramphenicol, 100 μg ml −1 ampicillin, 0.8% glucose and 200 ng ml −1 AHT at 32 °C. Samples were taken at an OD 600 of 0.5 and complementation was monitored by microscopy. AmiA overproduction and purification E. coli JM83 cells transformed with IBA2- amiACp were grown in no-salt LB in presence of 300 mM sucrose at 30 °C until they reached an OD 600 of 0.6 and induced by the addition of 200 ng ml −1 AHT. After 3 h of incubation at 30 °C, cells were harvested and purification was performed using the manufacturer’s (IBA, Germany) protocol for cleared lysates. OmpA cleavage was controlled by MS as described below. AmiA activity assay Remazol staining of E. coli W3110 PG sacculi and dye-release assays were performed as described previously with slight modifications [8] . Stained sacculi (20 μl) were incubated at 37 °C for 16 h with 4 μM AmiA in 200 μl 50 mM Hepes, pH 7.5, 20% dimethyl sulphoxide. In vitro activity assays using lipid II as a substrate were carried out in a final volume of 40 μl containing 4 μM purified protein, 2 nmol lipid II, 50 mM Tris, pH 7.5 and 5% dimethyl sulphoxide and incubated for 4 h at 37 °C. Reaction products were extracted with 40 μl of n -butanol/pyridine acetate (2:1 v/v, pH 4.2) and analysed by TLC and MS as described previously [13] and below, respectively. For TLC, silica was used as the stationary phase, whereas the mobile phase consisted of chloroform–methanol–water–ammonia carbonate (88:48:10:1). Spots were visualized by phosphomolybdic acid (PMA) staining. For penicillin inhibition assays, the AmpR resistance marker in the AmiA Cp expression vector was exchanged with CamR resistance marker. MS For reaction products 1 μl of the sample was placed onto a ground steel matrix assisted laser desorption ionization time-of-flight target plate and allowed to dry at room temperature (RT). Each sample was then overlaid with 1 μl of matrix (saturated solution of 6-Aza-2-thiothymine in 50% ethanol/20 mM diammonium citrate) and air dried at RT again. Spectra were recorded in the reflector negative mode on a biflex III mass spectrometer (Bruker Daltonik, Germany). For protein analysis, 2 μl of the sample were mixed with 2μl of 2% trifluoroacetic acid solution. After adding 2 μl of matrix solution (2,5-DHAP/DAC), this ternary mixture was pipetted up and down until crystallization started. The suspension (1 μl) was spotted onto an AnchorChip 600 target and allowed to dry at RT. The spectra were recorded in the linear positive mode on a biflex III mass spectrometer. How to cite this article: Klöckner, A. et al. AmiA is a penicillin target enzyme with dual activity in the intracellular pathogen Chlamydia pneumoniae . Nat. Commun. 5:4201 doi: 10.1038/ncomms5201 (2014).